Direct growth of single-crystalline III–V semiconductors on amorphous substrates The III–V compound semiconductors exhibit superb electronic and optoelectronic properties. Traditionally, closely lattice-matched epitaxial substrates have been required for the growth of high-quality single-crystal III–V thin films and patterned microstructures. To remove this materials constraint, here we introduce a growth mode that enables direct writing of single-crystalline III–V’s on amorphous substrates, thus further expanding their utility for various applications. The process utilizes templated liquid-phase crystal growth that results in user-tunable, patterned micro and nanostructures of single-crystalline III–V’s of up to tens of micrometres in lateral dimensions. InP is chosen as a model material system owing to its technological importance. The patterned InP single crystals are configured as high-performance transistors and photodetectors directly on amorphous SiO 2 growth substrates, with performance matching state-of-the-art epitaxially grown devices. The work presents an important advance towards universal integration of III–V’s on application-specific substrates by direct growth. Owing to their high-electron mobilities and direct band gaps, III–V compound semiconductors are ideal for many electronic and optoelectronic applications such as high-performance transistors [1] , [2] , [3] , photovoltaics [4] , [5] , LEDs [6] and photodetectors [7] . The development of epitaxial growth techniques such as molecular beam epitaxy [8] , metal-organic chemical vapour deposition (MOCVD) [9] and pulsed laser deposition [10] have enabled the growth of single-crystalline III–V thin films with excellent performance for device applications. In order to obtain such high-quality single-crystalline thin films, the growth must be done on a closely lattice-matched substrate [11] . The growth of single crystals onto amorphous substrates would further enable new applications, such as providing a simplified pathway for heterogeneous integration of III–V devices onto application-specific substrates. However, deterministic synthesis of single-crystalline semiconductors on amorphous substrates presents a fundamental challenge in the field of materials science—one that arises from the thermodynamics and kinetics of nucleation and crystal growth. Specifically, the slow kinetics governing coalescence of two grains into a single grain dictates that any single-crystalline structure on an amorphous substrate must be grown from a single nucleus. Thus, for single-crystalline growth, the first nucleus that forms must grow to fill the desired volume before another nucleus is formed. Within most growth approaches, the relative nucleation and growth rates are difficult to control, and the maximum grain size attainable is often on the order of the material thickness, resulting in nanocrystalline structures for nanoscale thickness materials [12] . Because of the tremendous technology-driven need for single-crystalline semiconductors on amorphous substrates, a number of synthesis techniques have been explored in recent years. These approaches include (i) epitaxial growth of thin films on single-crystalline substrates followed by selective layer transfer to a desired substrate [2] , [4] , (ii) vapour–liquid–solid [13] , [14] , [15] , [16] , [17] , vapour–solid [18] , [19] or aerosol-based [20] nanowire growth. For GaN, in particular, the usage of ‘pre-orienting’ layers to conduct local hetero-epitaxy has also been demonstrated [21] , [22] . While such approaches have resulted in broadening the scope and functionality of various electronic materials with unique properties, direct growth of single-crystalline semiconductors with ‘user-defined’ geometries and dimensions on amorphous substrates has yet to be demonstrated. Such an approach would offer major advantages in terms of compatibility with traditional device processing technology, scalability and processing cost. In addition, it would provide a direct pathway to three-dimensional integration of electronic materials and devices with appreciable levels of complexity. Here, we introduce templated liquid-phase (TLP) crystal growth ( Fig. 1a ) as a synthetic approach for growth of high-performance, nano- and micro-scale single-crystalline compound semiconductors with user-defined geometries on arbitrary substrates. Indium phosphide is chosen as a model III–V material system owing to its importance in a wide variety of fields, from high-speed electronics to lasers and photovoltaics [5] , [7] , [13] , [23] . Thermally grown SiO 2 and glass are selected as examples of amorphous materials on which TLP crystal growth can be performed. 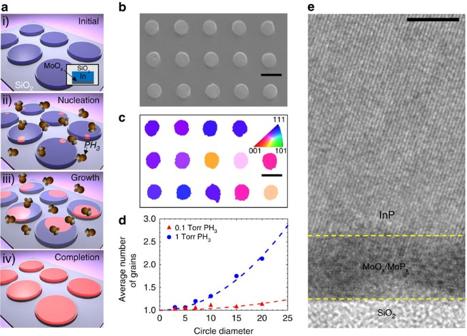Figure 1: Growth mechanism of single-crystalline InP. (a) Schematic of the process flow for TLP crystal growth. (b) SEM images of an array of 7 μm InP circles and (c) their corresponding EBSD maps. Scale bar, 10 μm. (d) The average number of grains per circle, measured via EBSD versus the circle diameter, showing a quadratic dependence. (e) TEM cross-sectional image of a portion of a patterned InP thin film showing the well-defined InP lattice on top of a MoOx/MoPxlayer on amorphous SiO2. Scale bar, 5 nm. Figure 1: Growth mechanism of single-crystalline InP. ( a ) Schematic of the process flow for TLP crystal growth. ( b ) SEM images of an array of 7 μm InP circles and ( c ) their corresponding EBSD maps. Scale bar, 10 μm. ( d ) The average number of grains per circle, measured via EBSD versus the circle diameter, showing a quadratic dependence. ( e ) TEM cross-sectional image of a portion of a patterned InP thin film showing the well-defined InP lattice on top of a MoO x /MoP x layer on amorphous SiO 2 . Scale bar, 5 nm. Full size image TLP growth and crystal quality For TLP growth of InP, indium metal is first lithographically patterned onto a Si/SiO 2 or glass substrate with a thin (1–10 nm) MoO x nucleation layer, and subsequently encapsulated by evaporated SiO x ( Supplementary Fig. 1 ). Growth is carried out in a low-pressure furnace at 500–535 °C in the presence of phosphine (PH 3 ) and H 2 . At the growth temperature, In is transformed into the liquid phase, but remains mechanically confined by the SiO x template. Phosphorous diffuses through the SiO x cap, and supersaturates the liquid In, precipitating out in the form of an InP nucleus. The key feature of this growth mode is that a phosphorous depletion zone forms around each growing nucleus, preventing further nucleation. Previously, we have shown that for continuous In thin films, this depletion zone can be on the order of hundreds of μm, leading to ultra-large grain sizes [24] , [25] . Here, we show that through pre-patterning the indium in mechanically confined templates such that the phosphorous depletion zone from the first nucleus occupies the entire template, ‘single crystalline’ InP growth in user-defined geometries can be achieved. Scanning electron microscope (SEM) images of the InP crystal arrays shaped into circles, rings and squares grown via TLP crystal growth are shown in Fig. 1b and Supplementary Fig. 2 . Critically, the original In template geometry is maintained after growth, allowing for deterministic shape control of InP crystals. The stoichiometry of the films is confirmed by electron dispersive spectroscopy (EDS) to be 1:1 In:P. X-ray diffraction spectroscopy on an array of InP circles ( Supplementary Fig. 3 ) displays only peaks corresponding to zincblende InP, indicating that all of the In has converted to InP. The crystallinity of the InP patterns with lateral dimensions of ∼ 5–7 μm is confirmed via electron backscatter diffraction (EBSD) mapping, showing that excluding twinning, each individual pattern is a single crystal but with different crystal orientations ( Fig. 1c , Supplementary Fig. 2 , Methods section, Supplementary Note 1 ). In addition, from the orientation distribution obtained from EBSD, it can be seen that there is a preferential texturing of the growth in the (1 0 n ) direction , where n ranges between 1 and 2 ( Supplementary Fig. 4 ). To study the effect of growth conditions and InP feature size on the number of grains, InP circles with diameters varying from 3 to 20 μm were patterned using TLP crystal growth at two different PH 3 partial pressures. From Fig. 1d and Supplementary Fig. 5 , it can be seen that the number of grains per circle increases according to a quadratic relation with the circle diameter, d , which can be fit by the equation: N grains is the average number of grains per circle and β is a proportionality factor that takes into account growth parameters such as P flux, the geometry associated with nucleation and the resulting average nucleation rate ( Supplementary Fig. 6 , Supplementary Note 2 ). As expected from our model, there is also a strong dependence of the number of grains on the PH 3 partial pressure. As the PH 3 partial pressure is lowered, the P flux into the liquid decreases, resulting in a reduced nucleation rate and larger P depletion zones ( Supplementary Note 2 ). This is reflected in a drop in β from 3 × 10 −3 to 4 × 10 −4 as the PH 3 partial pressure is reduced from 1 to 0.1 Torr, allowing the average number of grains per feature to be maintained at near unity even for diameters as large as 20 μm. Transmission electron microscopy (TEM) was used to examine the crystallinity of the InP patterns. From the cross-sectional TEM image of an InP sample shown in Fig. 1e , it can be seen that a crystalline InP lattice sits on top of the amorphous SiO 2 substrate with a thin MoO x /MoP x nucleation layer in between, clearly showing the non-epitaxial nature of TLP crystal growth. To demonstrate the versatility of the TLP crystal growth technique, the world’s smallest version of the ‘Lorem Ipsum’ placeholder text is written in crystalline InP lettering with a stroke width of 150 nm ( Fig. 2a ). In addition, a single-crystalline Berkeley ‘Cal’ logo with dimensions of 80 × 60 μm is shown in Fig. 2b with its structural, compositional and optoelectronic properties characterized via EBSD, EDS mapping and photoluminescence imaging ( Fig. 2c , Supplementary Fig. 7 ), respectively. While letters are used for demonstration purposes, the geometric degrees of freedom available to grow single-crystalline materials with TLP crystal growth are of great significance for the fabrication of practical electronic and photonic devices. 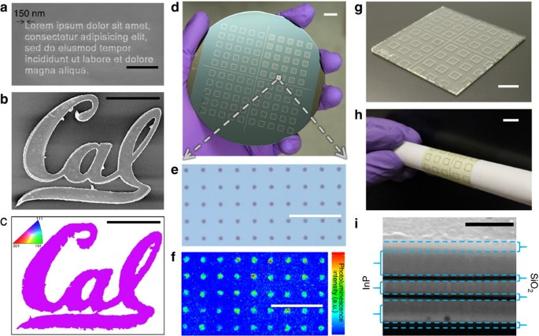Figure 2: Scalability and growth on ‘novel’ substrates. (a) SEM image of InP text with a linewidth of 150 nm. Scale bar, 3 μm. (b) An SEM image and corresponding (c) EBSD map of a single-crystalline UC Berkeley ‘Cal’ logo grown via TLP crystal growth. Scale bar, 30 μm. The Cal script logo is a federally registered trademark and may not be used without permission of The Regents of the University of California. (d) An optical image of a 4-inch Si/SiO2wafer patterned with arrays of 3 μm diameter InP dots located within each square InP box. Scale bar, 1 cm. (e) Zoomed in optical image of an array of dots on the wafer and (f) their corresponding photoluminescence image. Scale bar, 50 μm. (g) An optical image of patterned InP dots grown on a∼6 × 6 cm borosilicate glass slide. Scale bar, 1 cm. (h) An optical image of the patterned InP dot array transferred onto a PET substrate wrapped around a glass tube with a diameter of 1.5 cm. Scale bar, 1 cm. (i) Cross-sectional SEM image of three layers of InP grown with 30 nm of SiOxbetween each layer. Scale bar, 500 nm. Figure 2: Scalability and growth on ‘novel’ substrates. ( a ) SEM image of InP text with a linewidth of 150 nm. Scale bar, 3 μm. ( b ) An SEM image and corresponding ( c ) EBSD map of a single-crystalline UC Berkeley ‘ Cal ’ logo grown via TLP crystal growth. Scale bar, 30 μm. The Cal script logo is a federally registered trademark and may not be used without permission of The Regents of the University of California. ( d ) An optical image of a 4-inch Si/SiO 2 wafer patterned with arrays of 3 μm diameter InP dots located within each square InP box. Scale bar, 1 cm. ( e ) Zoomed in optical image of an array of dots on the wafer and ( f ) their corresponding photoluminescence image. Scale bar, 50 μm. ( g ) An optical image of patterned InP dots grown on a ∼ 6 × 6 cm borosilicate glass slide. Scale bar, 1 cm. ( h ) An optical image of the patterned InP dot array transferred onto a PET substrate wrapped around a glass tube with a diameter of 1.5 cm. Scale bar, 1 cm. ( i ) Cross-sectional SEM image of three layers of InP grown with 30 nm of SiO x between each layer. Scale bar, 500 nm. Full size image One major advantage of TLP crystal growth is ease of scalability. Unlike traditional III–V growth where both group III and V elements are introduced in the vapour phase, only the group V element is in the vapour phase, and the geometry is fixed by the template. This allows for simple reactor designs which can be easily scaled up to large scales. Furthermore, as growth only occurs when both group III and group V elements are present, the templates essentially provide a self-limiting growth mechanism, preventing unwanted thickness or compositional variation across a wafer. As a demonstration, Fig. 2d–f shows optical images as well as a corresponding photoluminescence image of arrays of InP circles outlined by InP bars, grown across a full 4-inch Si/SiO 2 wafer using a simple cold-wall furnace. The relatively low temperature required for TLP crystal growth also allows for a broad range of substrates upon which single-crystalline III–V’s can be grown. As an example, InP circles were directly written onto a borosilicate glass slide ( Fig. 2g ) and their optical quality was verified via photoluminescence imaging ( Supplementary Fig. 8 ). In addition, the grown InP can be fully transferred onto plastic substrates for applications where a flexible substrate is desired. As an example, Fig. 2h and Supplementary Fig. 9 , show an optical image and the corresponding photoluminescence image, respectively, of the InP circle arrays transferred onto a polyethylene terephthalate (PET) substrate using polyamic acid [26] . A unique feature of the TLP crystal growth process is that complex 3D architectures can be achieved, beyond the limits of traditional processes. For instance, multilayers of InP single crystals separated by amorphous SiO x layers can be grown in one cycle by starting with substrates consisting of multilayer In/SiO x layers, as demonstrated in the cross-sectional SEM image in Fig. 2i . This can have broad implications for future design of monolithic 3D electronics. In situ doping A critical component of semiconductor growth is the ability to tune the optical and electrical properties; in particular, the doping concentration. To explore this capability, GeH 4 gas was introduced into the growth chamber during growth to achieve controlled in situ n-type Ge doping of InP. 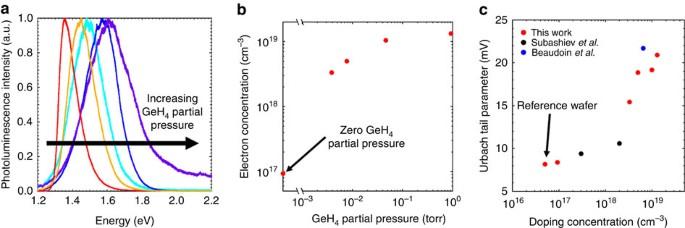Figure 3:In situdoping. (a) Photoluminescence spectra of five InP samples grown with GeH4pressures of 0, 3.9, 7.7, 46 and 900 mTorr of GeH4. As the GeH4partial pressure is increased, the peak of the photoluminescence spectra blue-shifts, signifying higher electron concentrations. (b) A plot of the electron concentration, approximated from the peak position of the photoluminescence spectra using the Burstein–Moss effect, as a function of the GeH4partial pressure. (c) The Urbach tail parameter is plotted versus the approximated doping level showing that the crystal quality is on par with that of single-crystalline wafers/films at different levels of doping. Figure 3a shows the normalized photoluminescence spectra of InP single crystals grown under different partial pressures of GeH 4 . Significant blue-shifting of the photoluminescence peak versus a lightly doped reference wafer ( Supplementary Fig. 10 ) is observed as the GeH 4 partial pressure is increased owing to the Burstein–Moss effect, indicating increased electron concentrations [27] , [28] , [29] . The electron concentrations, approximated from the photoluminescence peak energies (see Methods section), are plotted versus the GeH 4 partial pressure in Fig. 3b indicating that TLP grown InP can be doped up to a degenerate level of ∼ 1.3 × 10 19 cm −3 , near the upper limit of electron doping in InP [30] . From the photoluminescence spectra, the Urbach tail parameter is also extracted and plotted versus the carrier concentration level in Fig. 3c (ref. 31 ). The Urbach tail parameter is an important figure of merit regarding the band edge sharpness arising from crystal defects, thermal vibrations and charged impurities [32] , [33] . As can be seen, the Urbach tails of our non-epitaxial TLP grown samples are similar to the values reported in literature for InP single crystal wafers at various respective levels of doping [34] , [35] . Figure 3: In situ doping. ( a ) Photoluminescence spectra of five InP samples grown with GeH 4 pressures of 0, 3.9, 7.7, 46 and 900 mTorr of GeH 4 . As the GeH 4 partial pressure is increased, the peak of the photoluminescence spectra blue-shifts, signifying higher electron concentrations. ( b ) A plot of the electron concentration, approximated from the peak position of the photoluminescence spectra using the Burstein–Moss effect, as a function of the GeH 4 partial pressure. ( c ) The Urbach tail parameter is plotted versus the approximated doping level showing that the crystal quality is on par with that of single-crystalline wafers/films at different levels of doping. Full size image Electronic characterization The electronic quality and practical utility of TLP-growth InP in the shape of microwires (μWires) were explored by fabricating long-channel Schottky n-type metal-oxide-semiconductor field effect transistors (MOSFETs) with top gates ( Fig. 4a–c ). The transfer and output characteristics of an InP transistor on a Si/SiO 2 substrate with a gate length of 3 μm and body thickness of ∼ 125 nm are shown in Fig. 4d,e , respectively. The device exhibits an ON-current of 120 μA μm −1 at V GS = V DS =2 V with an ON/OFF current ratio of >10 5 and peak extrinsic transconductance of 100 S μm −1 , which is excellent for a long-channel device. An effective electron mobility of μ=675 cm 2 V −1 s −1 is extracted from device simulations (see Methods section), which compares favourably with unpassivated InP nanowire/microwire MOSFETs in literature [9] , illustrating the excellent electronic quality of the InP grown here. In addition, top-gated InP photo-MOSFETs were also fabricated on Si/SiO 2 substrates using the device structure above except that a transparent indium tin oxide (ITO) gate electrode is used with a channel length of L G =20 μm. The device electrical characteristics were measured under dark and under steady-state illumination from a bandpass filtered white light source with an optical intensity of 15.6 mW cm −2 . The device exhibits a strong photoresponse ( Fig. 4f ) with a peak responsivity of ∼ 700 A W −1 at V GS =3.4 V ( Fig. 4g ). Furthermore, the specific detectivity ( D *) of this device displays a maximum of ∼ 8.4 × 10 11 Jones at room temperature, comparable to state-of-the-art single-crystalline epitaxial InGaAs detectors [14] . 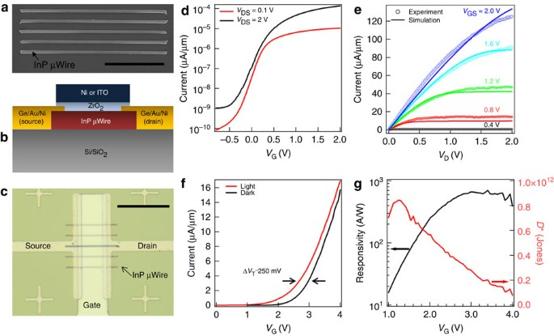Figure 4: Electronic characterization. (a) An SEM image of typical 1-μm wide InP μWires used for MOSFET fabrication. Scale bar, 20 μm. (b) A cross-sectional schematic of the InP MOSFETs along with (c) an optical image of a MOSFET with 5 μwires as the channel. Scale bar, 50 μm. (d) The transferIDS-VGSand (e) outputIDS-VDScurves of an InP transistor with a single μWire as the channel and a 3 μm gate length. (f) The transfer characteristics of a photo-MOSFET in dark and exposed to 15.6 mW cm−2of light, showing a large threshold voltage shift of∼250 mV. (g) The responsivity and detectivity of the photo-MOSFET are plotted versus the gate voltage bias. Figure 4: Electronic characterization. ( a ) An SEM image of typical 1-μm wide InP μWires used for MOSFET fabrication. Scale bar, 20 μm. ( b ) A cross-sectional schematic of the InP MOSFETs along with ( c ) an optical image of a MOSFET with 5 μwires as the channel. Scale bar, 50 μm. ( d ) The transfer I DS - V GS and ( e ) output I DS - V DS curves of an InP transistor with a single μWire as the channel and a 3 μm gate length. ( f ) The transfer characteristics of a photo-MOSFET in dark and exposed to 15.6 mW cm −2 of light, showing a large threshold voltage shift of ∼ 250 mV. ( g ) The responsivity and detectivity of the photo-MOSFET are plotted versus the gate voltage bias. Full size image In conclusion, we have demonstrated a technique that enables direct ‘writing’ of optoelectronic-quality single-crystalline III–V semiconductors on amorphous substrates. The elimination of the requirement for lattice-matched substrates as well as the improved scalability of this growth mode enables ubiquitous integration of III–V semiconductors for a wide range of applications on user-defined substrates. While InP was used as a model growth system in this work, the TLP crystal growth method is one that, from a thermodynamic and kinetic point of view, is expected to be applicable to other technologically important III–V’s. As an example, proof of concept demonstrations using the TLP process to grow GaP and InSb are shown in Supplementary Fig. 11 . In addition, single crystals grown via the TLP growth process may potentially be utilized as a virtual substrate in epitaxial growth processes, allowing for the realization of high-quality semiconductor heterostructures grown directly onto amorphous substrates. Future work on control of crystal orientation of individual patterns may further extend the tunability of the TLP growth mode, for instance, by making nucleation of a specific orientation thermodynamically favourable through surface engineering of the nucleation layer or via the introduction of geometric constraints using principles from graphoepitaxy [12] . Patterning and growth of InP First, a clean Si wafer with a 50-nm thick thermal oxide was lithographically patterned with the desired InP shape ( Supplementary Fig. 1a ). For the glass sample in Fig. 2g , a borosilicate glass slide was patterned instead. A thin 1–10 nm thick MoO x layer was evaporated ( Supplementary Fig. 1b ) followed by evaporation of In of the desired thickness and a 10–100-nm thick SiO x layer ( Supplementary Fig. 1c ). As SiO 2 has a high surface energy for nucleation [24] , the MoO x layer helps to promote nucleation of the InP [25] . To obtain a smooth In film, the evaporation of the In and SiO x bilayer was done with the substrate chuck cooled to <150 K using liquid N 2 . The whole MoO x /In/SiO x stack was then lifted off ( Supplementary Fig. 1d ). After liftoff, angled evaporation was utilized to coat the exposed side regions of the In with SiO x with thicknesses ranging from 4 to 50 nm ( Supplementary Fig. 1e,f ). During the growth, the SiO x template confines the liquid In so that the resulting InP crystal has the same shape as that of the original In pattern. Growth of the InP patterns for EBSD crystal analysis and transistors were carried out in a hot-wall CVD tube furnace. In all, 10% PH 3 in H 2 was used as the phosphorous source and was further diluted to the desired dilution. Growth of the 4-inch wafer, sample on glass and doping-dependent studies were done in a cold-wall CVD system. In all, 10% GeH 4 in H 2 was used as the Ge dopant source. The samples were grown for 10–20 min at pressures of 100–300 Torr (partial PH 3 pressure of 0.1–10 Torr) and growth temperatures ranging between 500 and 535 °C. EBSD characterization EBSD characterization was carried out in an FEI Quanta SEM with an Oxford Instruments EBSD detector. Analysis of the maps were done by the Oxford Aztec and Tango software programs. Orientation maps were generated and plotted using the inverse pole figure colour scheme. Twin boundary removal was done by ignoring the <111> 60° rotational boundaries within the crystals and plotting the surface orientation of each grain. Photoluminescence spectra and imaging Photoluminescence spectra were taken by a HORIBA LabRAM HR800 tool with a 532 nm excitation wavelength. For photoluminescence imaging, a red LED was used as the excitation light source and images were taken by an Andor silicon CCD camera through an optical microscope with a GaAs wafer used to filter out the irradiation wavelengths. Electron concentration extraction The electron concentration, n , can be approximated using the equation [27] : where ΔE is the shift of the photoluminescence peak energy from an undoped reference (1.34 eV taken from a 5 × 10 16 cm −3 doped reference wafer, Supplementary Fig. 10 ) and m/m 0 is the ratio of the effective electron mass of InP to the free electron mass. Urbach tail fitting The absorption at the band edge, is related to the photoluminescence spectra by the van Roosbroeck–Schockley equation by [27] where P(v) is the photoluminescence intensity as a function of frequency v , h is Planck’s constant, and k T is the thermal energy (25.6 mV at room temperature). E 0 , the slope at the absorption band edge, is the Urbach tail parameter, which describes the sharpness at the band edge and is a good indicator of crystal and optoelectronic quality. Device fabrication InP microwires with dimensions of 1 × 50μm and thickness of 125 nm were grown using TLP crystal growth as described above. Photolithography was used to lithographically define the source/drain contacts followed by evaporation of 3/10/40 nm of Ge/Au/Ni and liftoff. The source/drain contacts were subsequently annealed at 375 °C for 5 min to alloy the Ge with InP in the contact regions to improve contact resistance. In all, 10 nm of ZrO 2 was then deposited via atomic layer deposition at a temperature of 200 °C. Finally, photolithography was used once again to define the gate electrode. For the MOSFETs, 40 nm of Ni was evaporated as the top gate metal while for the photo-MOSFETs, 30 nm of ITO was deposited via sputtering instead to allow optical access to the channel. Sentaurus simulations Detailed semi-classical drift-diffusion simulations were carried out utilizing the Sentaurus Device simulator to accurately model the device performance. The parameter extraction was carried out by first matching the subthreshold region (−0.2 V< V GS <0.15 V) utilizing InP/ZrO 2 surface interface traps and gate work function as the fitting parameters and performing a least squares error fit, enabling accurate simulation of the mobile charge versus gate voltage. The mobility and series resistance of the device were extracted by minimizing the least squares error for all the I DS - V DS curves (0 V< V DS <2 V) for V GS =0.4, 0.8, 1.2, 1.6 and 2 V simultaneously. How to cite this article: Chen, K. et al. Direct growth of single-crystalline III–V semiconductors on amorphous substrates. Nat. Commun. 7:10502 doi: 10.1038/ncomms10502 (2016).